Integrated redox-active reagents for photoinduced regio- and stereoselective fluorocarboborylation Vinylboronates and alkylboronates are key components in variegated transformations in all facets of chemical science. The synthesis of vinylboronates and alkylboronates suffers from step-tedious and poor stereoselective procedures. We have developed a regulated radical difunctionalization strategy for the construction of fluorine-containing vinylboronates and alkylboronates with an integrated redox-active reagent IMDN-SO 2 R F . This bench-stable imidazolium sulfonate cationic salt offers a scalable and operational protocol for the fluoroalkylation-borylation of unsaturated hydrocarbons in a high regio- and stereoselective manner. The products can be further transformed into valuable fluorinated building blocks. Difunctionalization of alkenes and alkynes has been widely explored for rapid diversification of double/triple bonds [1] , [2] , [3] , [4] , [5] , [6] . Traditional transition metal-catalyzed difunctionalization methods have been well-developed to control the regioselectivity and stereoselectivity [7] , [8] . Along these lines, cascade radical addition of unsaturated hydrocarbons in the absence of metallo-intermediate has been realized through careful manipulation of the radical reactivities [9] , [10] , [11] . A single process to achieve radical difunctionalization with extensive functionality tolerance, especially fluorine-containing moieties, is of great value in altering the physical and biological properties of the unsaturated hydrocarbons [4] , [12] , [13] , [14] , [15] , [16] , [17] , [18] . Studer and co-workers [19] have reported a radical 1,2-trifluoromethylboration of unactivated alkenes using gaseous CF 3 I. Meanwhile, the direct 1,2-fluoroalkylboration of alkynes has also been explored [20] , [21] , [22] . The consequential vicinial vinylboronates, which can be readily transformed to a myriad of fluorine-containing building blocks, have been seldom realized. The only two existing approaches of trifluoromethylated vinylboronates were derived from fluorinated alkynes [23] and oxiranes [24] . The inaccessibility of those pre-functionalized precursors and operationally tedious procedures prohibited the stepwise fluorination-borylation strategies from practical use (Fig. 1a ). Thus, the development of regioselective installation of fluoroalkyl and boronated functionalities to unactivated hydrocarbons in the absence of transition-metal catalysts represents great challenge. Fig. 1: Origin of the reaction design. a Early reports on borylation of CF 3 -containing substrates. b Lewis base-activated radical borylation. c The design for dual functional redox-active reagent. d Imidazolium sulfonate-derived bench-stable fluoroalkylating reagent. e Mechanistic insight of sequential radical trifluoromethylborylation. Full size image Due to the complexity of radical process incorporating C–C and C–B bonds formation, several issues need to be addressed, including the reactivities of carbon and boron-centered radicals, the regioselectivity of the radical additions to unsymmetrical alkynes, and stereoselectivity towards E / Z vinylboronates. Typically, a radical borylation process [25] , [26] , [27] , [28] , [29] , [30] , [31] , [32] often employs Lewis basic solvents/mediators such as DMAc [33] , [34] , DMF [19] , [35] , phthalimide [36] , and pyridine [37] , [38] for the activation of diboron reagents via homolytic cleavage of B–B bonds (Fig. 1b ). However, the exogenous Lewis base-activated diboron species inevitably deplete CF 3 radicals that generated promptly from the trifluromethylating reagents, unable to engage in the desired trifluoromethylborylation sequence (for DFT calculation details, see Supplementary Fig. 18 ). Inspired by recent radical-induced difunctionalization strategies [39] , [40] , we intend to design an integrated reagent that progressively releases CF 3 radical for alkene/alkyne addition, and the endogenous Lewis basic residue subsequently activates the B–B bond for further borylation (Fig. 1c ). Trifluoromethanesulfinate-derived fluorinating reagents have been devised and adopted for direct functionalization of alkenes, alkynes, and arenes [41] . In contrast, the highly hydroscopic and corrosive trifluoromethanesulfonic anhydride (Tf 2 O) as a trifluoromethyl source is rarely explored. For its strong electrophilic nature, triflic anhydride is commonly used as an alcohol and amine protecting agent [42] , [43] , [44] . Qing and co-workers [45] have described a triflated pyridine intermediate (Tf − Py + ·OTf − ) that generated in situ for trifluoromethylated arenes and alkynes. However, the strong electron-withdrawing triflate-derived pyridinium complex is preferably dissociated and unattainable in solid or liquid phase. We speculated that a more basic N- heterocycle such as imidazole could harness the highly reactive Tf 2 O to assemble a bench-stable redox-active reagent. The positive charge of the resulting imidazolium trifluoromethanesulfonate can be delocalized on both nitrogen. Through the cleavage of the stabilized N–S bond (BDE ≈ 70 kcal mol −1 ) [46] , this cationic complex undergoes SET process to generate CF 3 SO 2 radical. Meanwhile, as a Lewis base, the imidazole residue can further activate the diboron reagents towards homolytic cleavage of the diboron reagent [20] , [34] , [35] , [36] , [37] , [38] , [39] . Herein, we have synthesized a dual functional reagent IMDN-SO 2 CF 3 1a–1g , a scalable and air-stable crystalline salt for a sequential radical fluoroalkylation-borylation of unsaturated hydrocarbons (Fig. 1d ). First, under the irradiation, Ir(III)* can reduce the cationic reagent 1 to a neutral radical I and releases CF 3 radical, SO 2 , and imidazole. Then the addition of ·CF 3 to the alkyne regioselectively furnishes vinylic radical II . Subsequent addition of vinyl radical II to B 2 cat 2 affords a Z -vinyl diboron radical III . The control of stereoselectivity is governed by steric repulsion between the trifluoromethyl group and the boronates. The following activation of diboron by the Lewis basic imidazole forms a highly reactive B–N heteroleptic intermediate IV , which leads to the carboborylation product 3 and imidazole-stabilized boryl radical V . Finally, photo-oxidation of V followed by coupling with − OTf affords boryl imidazolium salt VI and regenerates Ir(III) (Fig. 1e ). These proposed intermediates and selectivities are supported by DFT calculations (see Supplementary Figs. 16–19 ) This photoinduced cascade radical difunctionalization offers a concise and applicable protocol for constructing highly regio- and stereoselective fluorine-substituted vinylboronates and vicinal fluoroalkyl boronates. 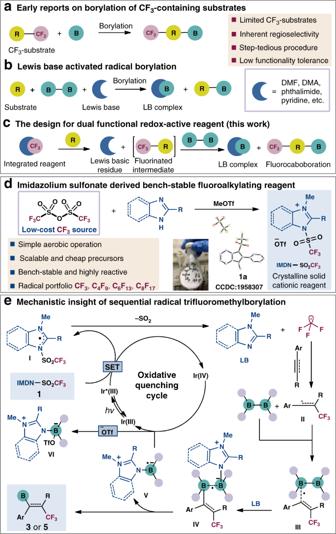Fig. 1: Origin of the reaction design. aEarly reports on borylation of CF3-containing substrates.bLewis base-activated radical borylation.cThe design for dual functional redox-active reagent.dImidazolium sulfonate-derived bench-stable fluoroalkylating reagent.eMechanistic insight of sequential radical trifluoromethylborylation. Reaction optimization To validate the above hypothesis, we selected phenylacetylene ( 2a ) as pilot substrate to test the trifluoromethylborylation reaction (Table 1 ). After extensive screening of conditions (see Supplementary Tables 1 and 2 ), we found that when using 2.5 equivalents of IMDN-SO 2 CF 3 ( 1a ) ( E 1/2 red = −1.385 V vs SCE), 2 mol% of fac -Ir(ppy) 3 ( E 1/2 IV/III* = −1.73 V vs SCE) [47] , 2.5 equivalents of B 2 cat 2 in a mixed solvent of MeCN and EtOAc (1:3 v/v) at room temperature under the irradiation of 30 W blue LEDs, the vinylboronate product 3a could be obtained in 82% yield (determined by 19 F NMR) with over 20:1 Z / E ratio. Different imidazolium sulfonate reagents 1b – 1h were then examined (Table 1 ). The yield of 3a descended when the benzoimidazolium reagents 1b and 1c were used (entries 2 and 3). The counterion was found to be important for this transformation, as evidenced by the low yield (53%) obtained when using BF 4 − salt ( 1d , entry 4). The reaction proceeded with 2-phenylimidazole reagents 1e and 1f in 76% and 60% yield, respectively (entries 5–6). The dimethylated reagent 1g resulted in a lower conversion (entry 7). The electroneutral reagent 1h failed to produce the desired product under irradiation, which may due to the low reduction potential ( E 1/2 red = −1.808 V vs SCE) (entry 8). This result validated the precedential presumption that the cationic reagent can serve as a better electron acceptor to furnish N -centered neutral radicals [48] , [49] , [50] , [51] . Other diboron reagents, such as bis(pinacolato)diboron (B 2 pin 2 ) and bis(neopentylglycolato)-diboron (B 2 neop 2 ), did not provide the corresponding borylated products (entries 9–10). Addition of excess bases such as imidazole and pyridine resulted in much lower yields (entries 11–12). Table 1 Optimization of the reaction conditions. Full size table Substrate scope with respect to the alkynes Using 2 mol% of fac -Ir(ppy) 3 , IMDN-SO 2 CF 3 ( 1a ) (2.5 equiv), and B 2 cat 2 (2.5 equiv) at ambient temperature, a range of alkyens underwent fluoroalkylation-borylation with good efficiency. As shown in Fig. 2 , the reaction can be performed at a gram scale to give 3a in 61% yield and high stereoselectivity. Aromatic alkynes with electro-donating or electro-withdrawing substituents afford the desired products 3b – 3j in good to excellent yields (60–93%) with high regio- and stereoselectivity ( Z : E > 20:1). Fig. 2: Substrate scope of the alkynes. a Crude yields determined by 19 F NMR spectroscopy using benzotrifluoride or trifluoromethoxybenzene as an internal standard. b Values in parentheses are of isolated yields. c The E / Z ratio was determined by 19 F NMR. d The E / Z ratio was determined by 1 H NMR. e Crude yields determined by 1 H NMR spectroscopy using dibromomethane as an internal standard. f 2.0 mmol of 2p was used. Full size image Functionalities including halides ( 3b , 3m , 3n ), nitrile ( 3d ), ester ( 3g ), and boronate ( 3j ) are tolerated. Naphthyl- and thienyl-substituted alkynes also readily transformed into the Z -products 3h and 3i in good yields. The reaction could also be applied to alkynyl deuterium to produce the ( Z )-selective deuterated vinylboronates 3k – 3n in 52–72% yields. An attempt of more challenging internal alkyne substrate resulted in the tetrasubstituted olefin in high regio- and stereoselectivity ( 3o , 45%). For further investigation of the reaction scope, different fluoroalkylating reagents 1i – 1l have been synthesized and applied to the standard cabonborylation conditions. Perfluoro-butyl ( 1i ), hexyl ( 1j ), and octanyl ( 1k ) reagents could furnish the corresponding products 3q – 3s in good yields (81–87%). Using a perhalogenated ether-derived sulfonate ( 1l ), the vinylboronate 3t was formed in high yield. To demonstrate the scalability of such radical carboborylation protocol, the reaction was carried out on 10 mmol scale to afford 3a in 61% yield with equally high Z / E ratio. Under the standard reaction conditions, alkyl-substituted alkynes could not transform to the desired products. DFT calculations illustrate that the energy barrier of CF 3 radical addition to aliphatic alkynes is higher than that to aromatic alkynes. Furthermore, a competing pathway of CF 3 radical addition to B 2 cat 2 leads to other trifluoromethylated products. Therefore, an excess amount of alkyl alkyne substrate is needed to facilitate the main reaction pathway. By using four equivalents of the alkyne, the borylated product 3p can be obtained in 26% yield. For internal aliphatic alkynes, the computed barrier with the CF 3 radical is much higher than that for the reaction of B 2 Cat 2 with the CF 3 radical. Therefore, no desired product is obtained using internal aliphatic alkynes as substrate. Substrate scope with respect to the olefins The α -fluoroalkylated boronates are also useful fluorine-containing synthons for further elaboration. By slight variation of the standard reaction conditions (see Supplementary Tables 3 – 10 ), we have extended this carbonborylation protocol to a range of unactivated alkenes (Fig. 3 ). Using IMDN-SO 2 CF 3 ( 1e ), alkenes bearing ester and amide functionalities underwent radical 1,2-carbonboration to afford trifluoromethylated boronates ( 5a – 5h ) in good yields. Heteroaryl ( 5i – 5j ), sulfonyl ( 5k ), and oxygenated alkyl groups ( 5l – 5n ) at various positions of the alkenes were also found effective. Cyclic alkenes could also transform into the desired products 5q and 5y . Noteworthy, biorelevant molecules, such as boldenone, lanosterol, (+)- α -tocopherol, and estrone-derived terminal alkenes afforded β -trifluoromethylboronates ( 5r – 5u ) in good yields. Additionally, fluoroalkyl radicals including ·C 4 F 9 ( 1i ), ·C 6 F 13 ( 1j ), ·C 8 F 17 ( 1k ), and ·CF 2 CF 2 O(CF 2 ) 7 CF 2 Cl ( 1l ) were successfully stitched to unactivated olefins to afford fluoroalkylborylated products in moderate yields ( 5v – 5dd ). The reaction with styrene failed to afford the desired product due to inert reactivity of benzylic radical. Fig. 3: Substrate scope of the olefins. a Crude yields determined by 19 F NMR. b Values in parentheses are isolated yields. c The diastereomeric ratio determined by 1 H NMR. Full size image Synthetic applications The synthetic utility of the method was demonstrated in a number of transformations of the highly functionalized alkylboronates and alkenylboronates [20] , [52] , [53] (Fig. 4 ). Oxidation of β -CF 3 boronate 5a afforded hydroxylated product 6 in 62% yield. Silver-catalyzed radical deboronofluorination of 5a in aqueous solution provided the alkyl fluoride 7 in 76% yield. Vinylation, oxidative coupling, and homologation of 5p afforded functionalized products 8 – 10 in good yields. Halogenation of vinylboronic ester 3a resulted in the formation of β -CF 3 -vinyl bromide 11 (53%). Palladium-catalyzed Suzuki–Miyaura cross-coupling of 3a with (hetero)aryl iodides afforded the corresponding trisubstituted alkenes 12 (90%) and 15 (88%). 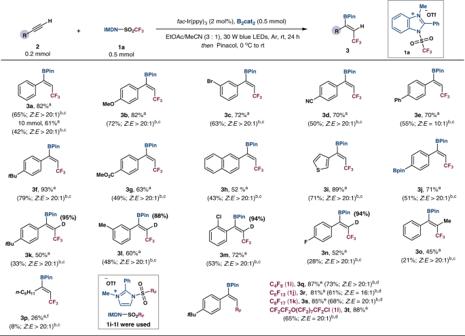Fig. 2: Substrate scope of the alkynes. aCrude yields determined by19F NMR spectroscopy using benzotrifluoride or trifluoromethoxybenzene as an internal standard.bValues in parentheses are of isolated yields.cTheE/Zratio was determined by19F NMR.dTheE/Zratio was determined by1H NMR.eCrude yields determined by1H NMR spectroscopy using dibromomethane as an internal standard.f2.0 mmol of2pwas used. Olefination and alkynylation using vinyl bromide or alkynyl bromide also proceeded smoothly to generate 13 and 14 in 73% and 96% yields, respectively. The coupling of 3a with bioactive estrone-derived triflate produced the corresponding product 16 with high stereoselectivity. Fig. 4: Further transformations. a H 2 O 2 (30%), NaOH (3 M), THF, 0 °C to rt. b Selectfluor, AgNO 3 , TFA, H 3 PO 4 , DCM/H 2 O, 50 °C. c Vinylmagnesium bromide, I 2 , THF, −78 °C to 0 °C. d n -BuLi, NBS, thiophene, THF, −78 °C. e n -BuLi, dibromomethane, THF, −78 °C to rt. f CuBr 2 , MeOH, 80 °C. g Pd(PPh 3 ) 4 (5 mol%), Cs 2 CO 3 , toluene, H 2 O, 80 °C. Full size image In summary, we have described an air-stable redox-active reagent IMDN-SO 2 R F 1 with high reactivity and scalability. A key design feature of this dual functional imidazolium sulfonate reagent is the cationic nature that favors the progressive formation of fluoroalkyl radicals by SET reduction under photocatalytic conditions. Meanwhile, the in situ-generated Lewis basic imidazole residue promotes the B–B bond cleavage. The integrated reagent is applicable to regulate the reaction sequence of carbon and boron-centered radicals to access various fluorine-bearing vinylboronates and alkylboronates with high stereo- and regioselectivities. Further study of this reagent is underway in our laboratory. General procedure for the synthesis of imidazolium salts 1 To a one-necked 1000 mL flask equipped with a magnetic stirrer, the corresponding imidazole (100 mmol), Et 3 N (150 mmol), and 600 mL DCM were added. The flask was then cooled in an ice bath, and 130 mmol (36.8 g) (CF 3 SO 2 ) 2 O was bubbled into the flask slowly. The mixture was stirred at room temperature for 2 h and evaporated in vacuo, quenched with water, and extracted with ethyl acetate (300 mL × 3). The combined organic layers were dried over Na 2 SO 4 , filtered, and concentrated. The product was purified by flash column chromatography on silica gel with n -pentane/ethyl acetate as eluent to give the imidazolyl sulfonamide. Under argon, to a solution of the imidazolyl sulfonamide in dried DCM (400 mL) was added dropwise MeOTf (or Me 3 OBF 4 ) (130 mmol) at 0 °C. Then, the mixture was stirred at room temperature for 12 h. (If EtOTf is used, the reaction is refluxed for 24 h.) After that, the mixture was concentrated under rotary evaporation to give a white solid (or a viscous liquid) crude product, to which Et 2 O (300 mL) was added. With vigorous stirring, a solid precipitate was formed and washed with Et 2 O (200 mL × 3) and dried in vacuo to yield the imidazolium salt 1 as a white solid. General procedure for the synthesis of vinylboronates 3 Under argon, to a solution of 1 (0.50 mmol, 2.5 equiv), B 2 Cat 2 (0.5 mmol, 2.5 equiv) and fac -Ir(ppy) 3 (2 mol%) in MeCN:EtOAc (1:3) (3 mL) was added corresponding alkynes 2 (0.2 mmol) at room temperature. After that, the tube was exposed to 30 W blue LEDs at room temperature about 30 h until the reaction was completed as monitored by TLC or GC-MS analysis. A solution of pinacol (236 mg, 2 mmol) in MeCN (1.0 mL) was added dropwise to the mixture at 0 °C. After 1 h, saturated ammonium chloride solution (15 mL) was added and the aqueous layer was extracted with hexane (3 × 15 mL). 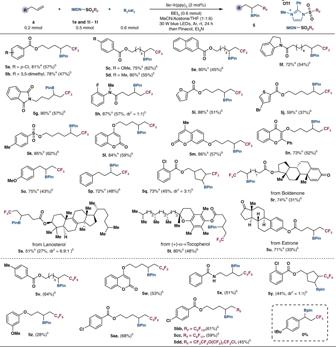Fig. 3: Substrate scope of the olefins. aCrude yields determined by19F NMR.bValues in parentheses are isolated yields.cThe diastereomeric ratio determined by1H NMR. 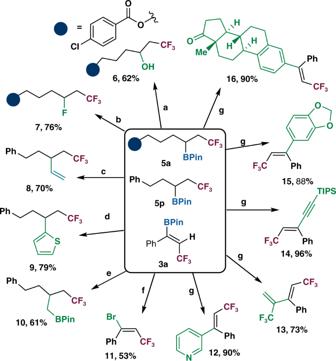Fig. 4: Further transformations. aH2O2(30%), NaOH (3 M), THF, 0 °C to rt.bSelectfluor, AgNO3, TFA, H3PO4, DCM/H2O, 50 °C.cVinylmagnesium bromide, I2, THF, −78 °C to 0 °C.dn-BuLi, NBS, thiophene, THF, −78 °C.en-BuLi, dibromomethane, THF, −78 °C to rt.fCuBr2, MeOH, 80 °C.gPd(PPh3)4(5 mol%), Cs2CO3, toluene, H2O, 80 °C. The combined organic layers were dried over Na 2 SO 4 , filtered, and concentrated. The product was purified by flash column chromatography on silica gel with n -pentane/ethyl acetate as eluent to give the vinylboronates 3 . General procedure for the synthesis of alkylboronates 5 Under argon, to a solution of 1 (0.50 mmol, 2.5 equiv), B 2 Cat 2 (0.6 mmol, 3.0 equiv) and fac -Ir(ppy) 3 (2 mol%) in 1:1 MeCN/acetone (0.2 mL) was added Et 3 B (0.6 mmol, 3.0 equiv, 1 mol/L in THF) and corresponding alkenes 4 (0.2 mmol) at room temperature. After that, the tube was exposed to 30 W blue LEDs at room temperature for 30 h until the reaction was completed as monitored by TLC or GC-MS analysis. A solution of pinacol (142 mg, 1.2 mmol) in Et 3 N (1.1 mL) was added to the mixture. After 1 h, the reaction mixture was evaporated in vacuo. The product was purified by flash column chromatography on silica gel with n -pentane/ethyl acetate as eluent to give the alkylboronates 5 .